A non-inactivating high-voltage-activated two-pore Na+channel that supports ultra-long action potentials and membrane bistability Action potentials (APs) are fundamental cellular electrical signals. The genesis of short APs lasting milliseconds is well understood. Ultra-long APs (ulAPs) lasting seconds to minutes also occur in eukaryotic organisms, but their biological functions and mechanisms of generation are largely unknown. Here, we identify TPC3, a previously uncharacterized member of the two-pore channel protein family, as a new voltage-gated Na + channel (Na V ) that generates ulAPs, and that establishes membrane potential bistability. Unlike the rapidly inactivating Na V s that generate short APs in neurons, TPC3 has a high activation threshold, activates slowly and does not inactivate—three properties that help generate long-lasting APs and guard the membrane against unintended perturbation. In amphibian oocytes, TPC3 forms a channel similar to channels induced by depolarization and sperm entry into eggs. TPC3 homologues are present in plants and animals, and they may be important for cellular processes and behaviours associated with prolonged membrane depolarization. Action potentials (APs) are the most fundamental electrical means that neurons use to communicate with each other. In mammals, neuronal APs generally last only a few milliseconds. This short period allows for energy conservation and a high capacity for information coding [1] . Beginning with the Hodgkin–Huxley studies of squid giant axon APs [2] , the functions and mechanisms underlying the generation of short APs have been extensively studied. All of the major ion channel proteins and genes responsible for initiating APs have been discovered, and many of them have been studied to atomic resolution [3] . There are nine plasma membrane voltage-gated Na + -selective channel (Na V ) pore-forming subunits (Na V 1.1–Na V 1.9) in mammals. These proteins have four homologous repeats of six transmembrane-spanning domains (4 × 6TM) [4] . The pores of voltage-gated K + channels (K V s) are made of four subunits of 1 × 6TM proteins [5] . The rapid inactivation of Na V s, within milliseconds, and the activation of K V s are responsible for the falling phase of APs and their short duration. Ultra-long AP-like depolarizations (ulAPs) that can last seconds to tens of minutes have also been recorded in many eukaryotic organisms, including unicellular amoebae [6] , [7] and multicellular organisms, such as algae [8] , Arabidopsis thaliana [9] , [10] , marine worms [11] , [12] , tunicates [13] and amphibians [14] , [15] . The functions of ulAPs are not well established, but they are thought to mediate ion homeostasis, cytoplasmic streaming, tissue repair, intercellular communication, response to environmental stimuli and polyspermy block [16] . The mechanisms underlying the generation of ulAPs are also poorly understood. In cells in low-ionic environments, such as pond water, Cl − efflux may mediate depolarization [8] , [17] . Many Cl − channels have been identified, but they have not been shown to generate long APs when introduced into heterologous expression systems [18] . Some ulAPs depend on a novel Na + channel on the plasma membrane [11] , [14] , [15] . The biophysical properties of this channel are markedly different from the rapidly inactivating Na V s. However, the molecular identity of the channel has not been verified. Here, we identify two-pore channel (TPC)3 as such a Na + -selective ion channel. TPC3 has a 2 × 6TM structure, half the size of the 4 × 6TM rapidly inactivating Na V s. TPC3 homologues are present in many different organisms that have been reported to have ulAPs. Unlike the 4 × 6TM Na V s, TPC3 has a high threshold voltage (~0 mV) for activation, and the channel does not inactivate. In fibroblasts and neurons transfected with TPC3, a brief depolarization stimulus elicits APs that last several seconds to minutes. When expressed in Xenopus oocytes, TPC3 forms an inducible voltage-gated Na + channel that does not inactivate and has an activity profile similar to that of the native conductance reported for a previously uncharacterized Na V . TPC3 is a plasma membrane-localized TPC family member To uncover the molecular mechanisms underlying the generation of ulAPs, we searched candidate proteins that can form non-inactivating Na V s. Previous studies have shown that plasma membrane Na V s can be formed by tetramers of 1 × 6TM proteins from the Na V Bac protein family in bacteria [19] and by monomers of 4 × 6TM proteins from the Na V family (Na V 1.1–Na V 1.9) in animals [20] , [21] . However, depolarizing holding potentials inactivate all members of these protein families. The third family of ion channels that has sequence similarity to the Na V Bac and Na V families is the TPC family of 2 × 6TM proteins, which has three vertebrate members (TPC1–3). TPCs are thought to function in intracellular organelles [22] , [23] . Whole-organelle patch-clamp experiments have shown that both native and heterologously expressed mammalian TPC1 and TPC2 create functional ion channels on endosomes and lysosomes [24] , [25] , [26] , [27] , [28] , [29] , [30] , [31] . TPC3 is the only one of the 25 proteins found in animals from the three ion channel families (1 × 6TM, 2 × 6TM and 4 × 6TM) with sequence similarities to Na V s and Ca V s that has not been electrophysiologically characterized. Humans and mice do not have a functional tpc3 gene [32] , [33] . Therefore, we isolated full-length TPC3 complementary DNA (cDNA) from zebrafish, Danio rerio (drTPC3). The sequence of drTPC3 is similar to human TPC1 (47% similarity and 23% identity), Na V s (46% similarity and 26% identity to hNa V 1.1) and Ca V s (43% similarity and 23% identity to hCa V 1.1). Interestingly, the S4 segments in the two repeats, IS4 and IIS4, have three charged residues (R/K) displaced in an every-third-residue fashion in their N-terminal regions, which is characteristic of voltage-gated channels, such as the Shaker K V channel ( Fig. 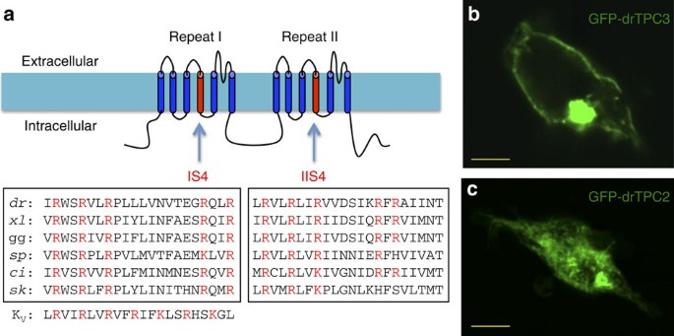Figure 1: TPC3 is expressed on the plasma membrane. (a) Upper: predicted membrane topology of TPC3s. Lower: sequences of IS4 and IIS4 of TPC3 proteins from zebrafish (Danio rerio, dr), frog (Xenopus laevis, xl), chicken (Gallus gallus, gg), sea urchin (Strongylocentrotus purpuratus, sp), tunicate (Ciona intestinalis, ci) and marine acorn worm (Saccoglossus kowalevskii, sk), aligned against the S4 region of the Shaker KVchannel. (b,c) Localization of N-terminally GFP-tagged drTPC3 (b) and drTPC2 (c) transfected into HEK293T cells. Scale bars, 5 μm. 1a ), Na V s and Ca V s. Figure 1: TPC3 is expressed on the plasma membrane. ( a ) Upper: predicted membrane topology of TPC3s. Lower: sequences of IS4 and IIS4 of TPC3 proteins from zebrafish ( Danio rerio , dr), frog ( Xenopus laevis , xl), chicken ( Gallus gallus , gg), sea urchin ( Strongylocentrotus purpu ratus, sp), tunicate ( Ciona intestinalis , ci) and marine acorn worm ( Saccoglossus kowalevskii , sk), aligned against the S4 region of the Shaker K V channel. ( b , c ) Localization of N-terminally GFP-tagged drTPC3 ( b ) and drTPC2 ( c ) transfected into HEK293T cells. Scale bars, 5 μm. Full size image In contrast to the intracellular localization of TPC1 and TPC2 (ref. 24 ), green fluorescent protein (GFP)-tagged drTPC3 was detected on the plasma membrane ( Fig. 1b ). As expected for many overexpressed membrane proteins, a weak GFP signal was observed on endolysosome-like organelles. Similar to mammalian TPC1s and TPC2s, Zebrafish TPC2 (drTPC2) was primarily localized to intracellular organelles ( Fig. 1c ). TPC3 forms a high-voltage-activated Na + channel As the electrophysiological properties of all other TPC members have been recorded from endolysosomes [25] , [26] , [27] , [28] , [29] , [30] , we first characterized drTPC3 expressed on endolysosomes using whole-endolysosomal recordings with symmetrical Na + concentration (145 mM) in the bath and pipette. Organelles expressing drTPC3 protein were identified by GFP fused to drTPC3. No obvious current was detected at voltages of −100 to +70 mV. When the voltage applied was increased above +70 mV, currents were detectable in a subset of GFP-positive endolysosomes (18/42, >100 pA at +150 mV; Supplementary Fig. 1 ). These results were in contrast to hTPC1- or hTPC2-expressing endolysosomes, which give robust currents under similar conditions [25] , [26] , [27] . In endolysosomes where a TPC3 current ( I TPC3 ) was detected, the current’s activation threshold of +70 mV was much higher than that of hTPC1 (~0 mV) under identical recording conditions (pH lumen 4.6) [26] and is unlikely to be reached by lysosomes under physiological conditions. To test whether drTPC3 formed a functional plasma membrane ion channel, we recorded whole-cell currents from HEK293T cells transfected with drTPC3. Little voltage-activated current was observed in HEK293T cells that were not transfected ( Fig. 2a ) or were transfected with the lysosome-localized drTPC2 ( Fig. 2b ). Remarkably, transfection with drTPC3, whether GFP-tagged ( Fig. 2c ) or untagged ( Fig. 2d ), generated robust currents elicited by a depolarizing membrane potential (14/15, >500 pA at +100 mV). 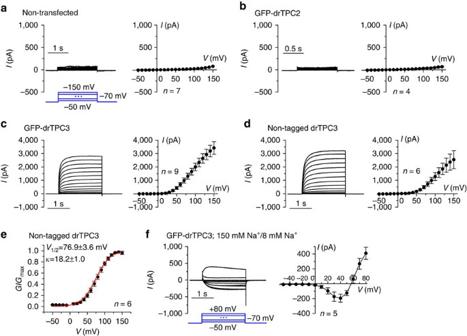Figure 2: TPC3 forms a high-voltage-activated plasma membrane Na+channel. (a–d) Whole-cell currents recorded with symmetrical [Na+] (150 mM) in the bath and pipette from nontransfected HEK293T cells (a), or cells transfected with GFP-tagged drTPC2 (GFP-drTPC2) (b), GFP-drTPC3 (c) or non-tagged drTPC3 (d). (e) Normalized conductance (G/Gmax)–voltage (V) relationships reconstructed fromd. (f) Similar to panelc, but recorded under asymmetrical [Na+] conditions (150 mM in the bath and 8 mM in the pipette). Left panels show representative traces obtained with a voltage-step protocol (shown inafora–d, and inf). Current (I)–voltage (V) relationships constructed using the current sizes at the end of the voltage steps are in right panels. Data are represented as mean±s.e.m. Figure 2: TPC3 forms a high-voltage-activated plasma membrane Na + channel. ( a – d ) Whole-cell currents recorded with symmetrical [Na + ] (150 mM) in the bath and pipette from nontransfected HEK293T cells ( a ), or cells transfected with GFP-tagged drTPC2 (GFP-drTPC2) ( b ), GFP-drTPC3 ( c ) or non-tagged drTPC3 ( d ). ( e ) Normalized conductance ( G / G max )–voltage ( V ) relationships reconstructed from d . ( f ) Similar to panel c , but recorded under asymmetrical [Na + ] conditions (150 mM in the bath and 8 mM in the pipette). Left panels show representative traces obtained with a voltage-step protocol (shown in a for a – d , and in f ). Current ( I )–voltage ( V ) relationships constructed using the current sizes at the end of the voltage steps are in right panels. Data are represented as mean±s.e.m. Full size image The drTPC3 was activated by depolarization ( Fig. 2d,e ) with slow kinetics ( Fig. 2c ; τ =224±35 ms at +50 mV). Under more physiological asymmetric Na + conditions (150 mM Na + in bath and 8 mM in pipette), drTPC3 generated an inward current at voltages from ~0 to 60 mV ( Fig. 2f ). The current–voltage ( I – V ) relationship was similar to that of other Na V s, but was right-shifted towards higher voltages. The channel’s activation threshold of ~0 mV was much higher than the activation threshold for 1 × 6TM and 4 × 6TM Na V s (approximately −50 to −40 mV [19] , [34] ). TPC3 does not inactivate The I TPC3 was not obviously inactivated at test voltages lasting as long as 20 s ( Fig. 3a–c ). In addition, pre-pulses of −100 to +150 mV, which have been shown to inactivate other plasma membrane Na V s at high voltages, did not cause steady-state inactivation of drTPC3 ( Fig. 3d,e ). The lack of obvious inactivation observed for TPC3 is unlike any of the other plasma membrane Na V s. Therefore, we conclude that drTPC3 forms a novel voltage-gated Na + channel with a high threshold for activation that does not inactivate. 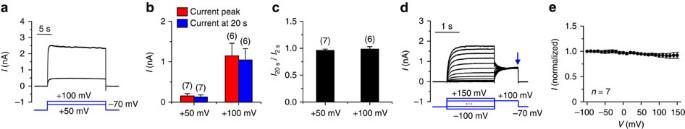Figure 3: TPC3 channels do not inactivate. (a) Representative whole-cell currents activated by 20-s-long step pulses to +50 and +100 mV (Vh=−70 mV). (b) Average amplitudes of the current peak and those at the end of pulses (20 s). (c) Current amplitudes obtained at the end of pulses normalized to those at the beginning (2 s). (d) Steady-state inactivation of TPC3. Currents were recorded with a test pulse to +100 mV following a pre-pulse of 2 s in duration, at voltages ranging from −100 to +150 mV (10-mV step). (e) Current amplitudes at the end of the test pulses (arrow ind) were plotted against pre-pulse voltages. Whole-cell currents were recorded from HEK293T cells transfected with drTPC3 (non-tagged). GFP-tagged drTPC3 generated similar non-inactivating currents (not shown; see alsoFig. 2). Numbers of cells are indicated in parentheses. Data are represented as mean±s.e.m. Figure 3: TPC3 channels do not inactivate. ( a ) Representative whole-cell currents activated by 20-s-long step pulses to +50 and +100 mV ( V h =−70 mV). ( b ) Average amplitudes of the current peak and those at the end of pulses (20 s). ( c ) Current amplitudes obtained at the end of pulses normalized to those at the beginning (2 s). ( d ) Steady-state inactivation of TPC3. Currents were recorded with a test pulse to +100 mV following a pre-pulse of 2 s in duration, at voltages ranging from −100 to +150 mV (10-mV step). ( e ) Current amplitudes at the end of the test pulses (arrow in d ) were plotted against pre-pulse voltages. Whole-cell currents were recorded from HEK293T cells transfected with drTPC3 (non-tagged). GFP-tagged drTPC3 generated similar non-inactivating currents (not shown; see also Fig. 2 ). Numbers of cells are indicated in parentheses. Data are represented as mean±s.e.m. Full size image TPC3 is Na + selective The sequence of drTPC3 is similar to those of the 4 × 6TM Ca V s and Na V s, but does not have an obvious sequence equivalent to the ‘DEKA’ or ‘EEEE’ ion selectivity-determining motif found in the pore-filter regions of the 4 × 6TM Na V s or Ca V s. Under conditions where the major cations were supplied by 150 mM Na + in the bath and 150 mM N -methyl- D -glucamine (NMDG) in the pipette, an inward I TPC3 could be elicited with depolarizing membrane potentials ( Fig. 4a ). However, replacing the Na + in the bath with 150 mM K + , 100 mM Ca 2+ or 150 mM NMDG + abolished the inward current, suggesting that drTPC3 was primarily permeable to Na + , but not to K + , Ca 2+ , Cl − or NMDG + ( Fig. 4a,b ). We used the reversal potentials measured under bi-ionic conditions to estimate the relative permeability of drTPC3 ( Fig. 4c,d ). The P Na / P Cs ratio was 88.1±14.5 ( n =6) and P Na / P K was 117.3±15.1 ( n =11). 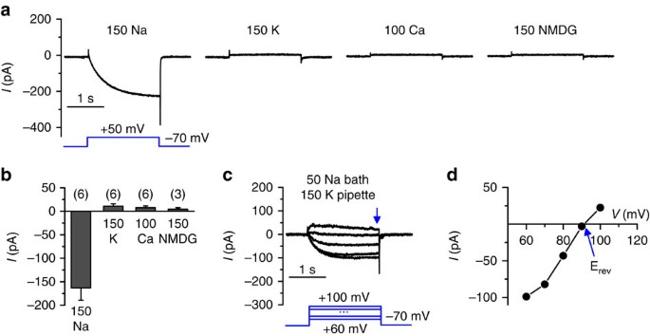Figure 4: TPC3 channels are Na+selective. Whole-cell currents were recorded from GFP-drTPC3-transfected HEK293T cells. Representative traces (a) and average amplitudes (b) of currents recorded with a pipette solution containing 150 mM NMDG+and bath containing 150 mM Na+, 150 mM K+, 100 mM Ca2+or 150 mM NMDG+as indicated. (c) Representative currents elicited by voltage pulses (illustrated) under bi-ionic condition (150 mM K+in pipette and 50 mM Na+in bath). (d) Current sizes obtained fromcplotted against test pulse voltages to obtain reversal potential (Erev) for the calculation of relative permeability. Data are represented as mean±s.e.m. The selectivity that TPC3 displayed for Na + was comparable to that of the 4 × 6TM Na V s. Figure 4: TPC3 channels are Na + selective. Whole-cell currents were recorded from GFP-drTPC3-transfected HEK293T cells. Representative traces ( a ) and average amplitudes ( b ) of currents recorded with a pipette solution containing 150 mM NMDG + and bath containing 150 mM Na + , 150 mM K + , 100 mM Ca 2+ or 150 mM NMDG + as indicated. ( c ) Representative currents elicited by voltage pulses (illustrated) under bi-ionic condition (150 mM K + in pipette and 50 mM Na + in bath). ( d ) Current sizes obtained from c plotted against test pulse voltages to obtain reversal potential ( E rev ) for the calculation of relative permeability. Data are represented as mean±s.e.m. Full size image I TPC3 was not inhibited by tetrodotoxin ( Fig. 5a,b ), a toxin that blocks several 4 × 6TM Na V s at concentrations in the sub-μM range. In contrast, drTPC3 was highly sensitive to inhibition by high-voltage-gated L-type Ca V inhibitors (Cd 2+ half-maximal inhibitory concentration (IC 50 ): 151±28 μM, Fig. 5c,d ; verapamil: 0.60±0.07 μM; Fig. 5e,f ; nifedipine: 3.35±0.26 μM, Fig. 5g,h ). 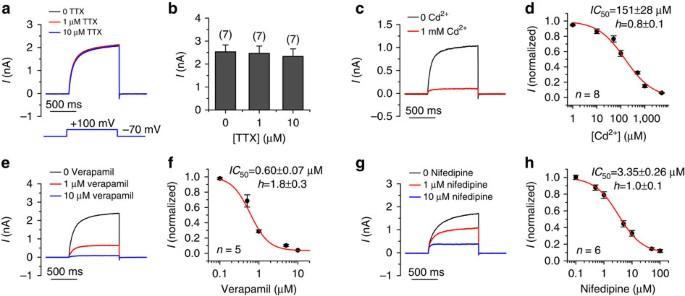Figure 5: TPC3 is insensitive to the NaVblocker tetrodotoxin (TTX), but is inhibited by CaVblockers. Whole-cell currents were elicited with a test pulse to +100 mV (Vh=−70 mV) and recorded under the symmetric [Na+] (150 mM in the bath and pipette) condition from GFP-drTPC3-transfected HEK293T cells. Inhibitors were added as indicated. Representative currents were recorded in the presence and absence of each drug. (a) Representative currents and (b) average current amplitudes in the presence or absence of TTX. (c) Representative currents and (d) dose response curve for Cd2+. (e) Representative currents and (f) dose response curve for verapamil. (g) Representative currents and (h) dose response curve for nifedipine. Current amplitudes normalized to that obtained without drug were fitted with the Hill equations. Data are represented as mean±s.e.m. Figure 5: TPC3 is insensitive to the Na V blocker tetrodotoxin (TTX), but is inhibited by Ca V blockers. Whole-cell currents were elicited with a test pulse to +100 mV ( V h =−70 mV) and recorded under the symmetric [Na + ] (150 mM in the bath and pipette) condition from GFP-drTPC3-transfected HEK293T cells. Inhibitors were added as indicated. Representative currents were recorded in the presence and absence of each drug. ( a ) Representative currents and ( b ) average current amplitudes in the presence or absence of TTX. ( c ) Representative currents and ( d ) dose response curve for Cd 2+ . ( e ) Representative currents and ( f ) dose response curve for verapamil. ( g ) Representative currents and ( h ) dose response curve for nifedipine. Current amplitudes normalized to that obtained without drug were fitted with the Hill equations. Data are represented as mean±s.e.m. Full size image TPC3 is insensitive to PI(3,5)P 2 and PI(4,5)P 2 PI(3,5)P 2 , a phosphatidylinositol bisphosphate enriched on endosomal and lysosomal membranes, potentiates several mammalian ion channels, including TRPM4, TRPMLs, TPC1 and TPC2 (refs 26 , 27 , 35 , 36 , 37 ). We measured I TPC3 from endolysosomes to test the sensitivity of TPC3 to PI(3,5)P 2 . Unlike hTPC1 and hTPC2 (refs 26 , 27 ), drTPC3 was not potentiated or inhibited by exogenous PI(3,5)P 2 ( Fig. 6a,b ). 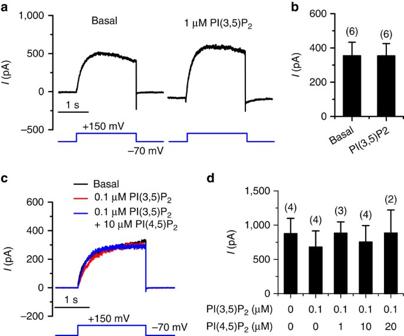Figure 6: TPC3 is insensitive to PI(3,5)P2and PI(4,5)P2. Endolysosomal currents were recorded from GFP-drTPC3-transfected HEK293T cells. Concentrations of PI(3,5)P2and PI(4,5)P2are indicated in the figure. (a) Representative current traces and (b) average current amplitudes in the absence (basal) or presence of PI(3,5)P2. (c) Representative current traces and (d) average current amplitudes in the absence or presence of PI(4,5)P2. Data are represented as mean±s.e.m. Figure 6: TPC3 is insensitive to PI(3,5)P 2 and PI(4,5)P 2 . Endolysosomal currents were recorded from GFP-drTPC3-transfected HEK293T cells. Concentrations of PI(3,5)P 2 and PI(4,5)P 2 are indicated in the figure. ( a ) Representative current traces and ( b ) average current amplitudes in the absence (basal) or presence of PI(3,5)P 2 . ( c ) Representative current traces and ( d ) average current amplitudes in the absence or presence of PI(4,5)P 2 . Data are represented as mean±s.e.m. Full size image In addition to requiring PI(3,5)P 2 for optimal activation, the endolysosome channel TRPML1 is inhibited by PI(4,5)P 2 (ref. 38 ), a plasma membrane-enriched lipid required for the normal functions of many ion channels [39] , [40] . TRPML1 activity is thought to be restricted to intracellular organelles, in part due to the opposing regulatory functions of PI(3,5)P 2 and PI(4,5)P 2 (ref. 38 ). In contrast to TRPML1, drTPC3 was not blocked by PI(4,5)P 2 , even at a concentration of 20 μΜ ( Fig. 6c,d ). As a control, we also tested the effects of PI(3,5)P 2 and PI(4,5)P 2 on the lysosome channel drTPC2. The drTPC2 was potentiated by PI(3,5)P 2 ( Supplementary Fig. 2a ) and inhibited by PI(4,5)P 2 ( Supplementary Fig. 2b ). The contrasting sensitivity to lipid regulation between TPC3 and other TPCs separates TPC3 from the endolysosome-confined channels. TPC3 supports ulAPs and bistability We used current-clamp recordings to test whether TPC3 supports the generation of ulAPs when transfected into HEK293T fibroblast cells. Without transfection, HEK293T fibroblasts are non-excitable and do not generate regenerative responses ( Fig. 7a , n =7). In the drTPC3-transfected cells, depolarizing stimuli, upon reaching a threshold of ~0 mV, elicited AP-like depolarizations that lasted seconds to many minutes (9/12, Fig. 7b–d ). Further increasing the stimulus strength sometimes ‘drove’ the membrane potential of the cell to a steady state of approximately +50 to +80 mV ( Fig. 7b ), close to the equilibrium potential of Na + (+91 mV). Interestingly, the cells remained at the newly established depolarized membrane potential until it was terminated by a hyperpolarizing pulse ( Fig. 7c ), a characteristic of cell membrane bistability. Thus, transfecting drTPC3 alone was sufficient to convert non-excitable cells into excitable ones. 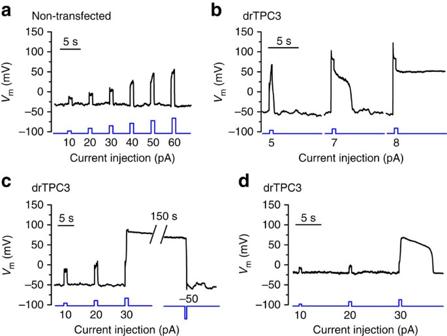Figure 7: TPC3 supports ultra-long action potentials and membrane bistability. Representative whole-cell current-clamp recordings were performed in HEK293T cells without (a) or with (b–d) GFP-drTPC3 transfection. Depolarizing current injection stimuli (illustrated below each recording with the sizes indicated) were applied. ulAPs were elicited from resting membrane potentials of −50 mV inbandc, or −20 mV ind. Figure 7: TPC3 supports ultra-long action potentials and membrane bistability. Representative whole-cell current-clamp recordings were performed in HEK293T cells without ( a ) or with ( b – d ) GFP-drTPC3 transfection. Depolarizing current injection stimuli (illustrated below each recording with the sizes indicated) were applied. ulAPs were elicited from resting membrane potentials of −50 mV in b and c , or −20 mV in d . Full size image We also tested the ability of TPC3 to support ulAPs and membrane bistability in mammalian neurons, which express high levels of K V s. In cultured mouse hippocampal neurons transfected with drTPC3, but not untransfected control neurons, a brief stimulus induced a long depolarization (4/18, Supplementary Fig. 3 ) and sometimes induced membrane bistability. TPC3 forms the Na + channel found in amphibian oocytes We next searched for a model system that is known to have a native Na + current similar to I TPC3 . Among the commonly studied cellular model systems, frog oocytes and eggs from Xenopus laevis and Rana pipiens generate ulAPs and are known to have a non-inactivating Na + channel activated at high voltages, whose molecular identity is unknown [14] , [15] . A peculiar but little-understood property of the native current in these models is its ‘induction’ by depolarization. A small current can be recorded from non-induced R. pipiens oocytes [15] , but robust currents in X. laevis oocytes can only be recorded after induction by a pre-pulse depolarization [14] ( Fig. 8a–c ). The native Xenopus oocyte channel had a high activation threshold, activated slowly and did not inactivate ( Fig. 8b,c ), similar to what has been previously reported [14] . The channel was inhibited by verapamil (IC 50 , 0.8 μM) and nifedipine (IC 50 , 7.19 μΜ) ( Supplementary Fig. 4 ). Thus, the biophysical and pharmacological properties of the unknown Xenopus channel are similar to those of drTPC3 expressed in HEK293T cells. 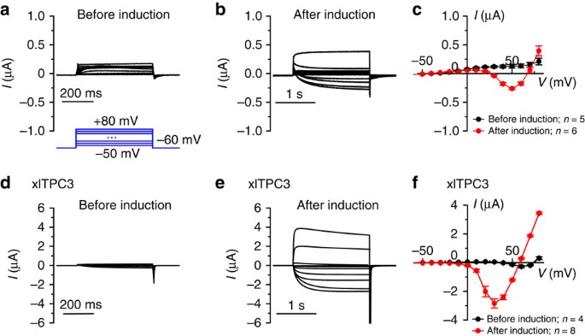Figure 8: TPC3-like current inXenopusoocytes. Two-electrode voltage-clamp recordings were performed withXenopusoocytes without (a–c) or with (d–f) xlTPC3 RNA injection. (a,b,d,e) Representative currents recorded with a voltage-step protocol (−50 to +80 mV with a 10-mV step,Vh=−60 mV, shown ina) before (a,d) and after (b,e) the oocyte was ‘induced’ with a 60-s depolarization of +50 mV. Capacitive transient currents are masked for clarity. (c,f) Average current–voltage relationships. Data are represented as mean±s.e.m. Figure 8: TPC3-like current in Xenopus oocytes. Two-electrode voltage-clamp recordings were performed with Xenopus oocytes without ( a – c ) or with ( d – f ) xlTPC3 RNA injection. ( a , b , d , e ) Representative currents recorded with a voltage-step protocol (−50 to +80 mV with a 10-mV step, V h =−60 mV, shown in a ) before ( a , d ) and after ( b , e ) the oocyte was ‘induced’ with a 60-s depolarization of +50 mV. Capacitive transient currents are masked for clarity. ( c , f ) Average current–voltage relationships. Data are represented as mean±s.e.m. Full size image To test whether the Xenopus oocyte Na + channel is encoded by TPC3, we cloned the full-length TPC3 homologue (xlTPC3) from X. laevis oocytes. xlTPC3 is highly similar to drTPC3 (57% identity, 75% similarity). When expressed in HEK293T cells, xlTPC3 formed a high-threshold voltage-activated Na + channel on the plasma ( Supplementary Fig. 5a,b ; n =5) and endolysosomal ( Supplementary Fig. 5c,d ; n =10) membranes. Similar to drTPC3, xlTPC3 was blocked by verapamil and Cd 2+ ( Supplementary Fig. 6 ). We then expressed xlTPC3 in its native environment by injecting xlTPC3 complementary RNA (cRNA) into Xenopus oocytes, and compared the properties of the resulting channel with those of the native one. In oocytes injected with xlTPC3 cRNA, but not in oocytes injected with H 2 O, a depolarizing pre-pulse induced a non-inactivating current that, compared with the native one, was increased by threefold 2 days after injection and 11-fold 7 days after ( Fig. 8d–f ). These data suggest that TPC3 forms the native Xenopus oocyte channel. We have identified the first high-voltage-activated, non-inactivating, Na + -selective plasma membrane ion channel and provided a molecular mechanism for the generation of ulAPs. These results and earlier extensive studies on short APs [2] , [3] , [41] make it clear that both short and ulAPs can be generated from voltage-gated Na + channels. The short APs are generated by rapidly inactivating Na V s, whereas the ulAPs are generated by non-inactivating Na V s. Cl − channels and slowly inactivating Ca V s may also generate APs lasting several seconds under certain conditions, which require further study. With the addition of TPC3 as a new family member, Na V s are now known to be formed by 1 × 6TM, 2 × 6TM and 4 × 6TM proteins, the three most likely combinations of 6TM channel pore-forming building blocks [42] . Like Ca V s, Na V s can also be divided according to their activation thresholds into low-voltage- and high-voltage-activated families. TPC3 is the only known high-voltage-activated Na V with an activation threshold of ~0 mV. The electrophysiological properties of all three members of the vertebrate TPC family have now been described. They all form Na + channels, with TPC1 and TPC3 being depolarization-activated [25] , [26] , [27] , [28] . In contrast to what was previously believed, the TPC family also forms plasma membrane ion channels. Thus, future studies addressing the physiology of TPC proteins should also include plasma membrane functions. In addition to their vastly different durations, there are other clear distinctions between short and ulAPs. For example, short APs can only be elicited from relatively negative resting membrane potentials because the Na V s are subject to steady-state inactivation at more depolarized voltages, even if still below the AP threshold. In contrast, ulAPs can be generated from much more depolarized membrane potentials ( Fig. 7d ) because TPC3 lacks steady-state inactivation. Short APs in mammalian neurons can also be induced by short weak depolarization stimuli, conditions achievable by synaptic inputs. The ulAPs, however, generally require much stronger stimuli with a longer duration of ~100 milliseconds. In frog oocytes, for instance, ulAPs are induced by a large depolarization of >0 mV or by sequential repetitive sub-threshold stimuli [14] , [43] . The egg ulAPs can also be activated by pricking the membrane or by sperm entry, mechanical or chemical stimuli that presumably lead to the membrane breaking and depolarization to ~0 mV for many milliseconds. A Ca V -mediated depolarization that lasts many milliseconds also precedes Na V opening in the ‘sperm-activated’ ulAPs in marine worm eggs [11] , [44] . If these ulAPs are indeed generated by TPC3, its slow activation kinetics and activation threshold close to 0 mV presumably explain the high stimulation threshold in terms of duration and amplitude for triggering the ulAPs. Because TPC3 activation can lead to a long-lasting large depolarization that sometimes does not repolarize, the high threshold for TPC3 activation may provide the cells with a low-pass filter mechanism that guards against unintended large variations in membrane potential caused by small changes in the environment. In practical terms, TPC3 and its derivatives with lower activation thresholds could serve as bistable switches for neuronal control when used in conjunction with channelrhodopsin [45] , [46] . Unlike short APs, the in vivo functions of ulAPs are largely unknown. The most well-studied ulAPs are observed in oocytes and eggs from several invertebrates and vertebrates [11] , [16] , [43] , [47] , which do not appear to have short APs. The long depolarization in some invertebrate eggs is proposed to mediate a fast electrical polyspermy block (but see also ref. 48 ). In frog oocytes and eggs under artificial conditions in a bath containing ~100 mM Na + , the ulAPs observed after electrical or mechanical induction appear to be dependent on a TPC3-like conductance [14] , [49] . However, it is unlikely that that the TPC3-like conductance is used to generate an electrical polyspermy block triggered by sperm entry. Under natural conditions, the eggs are fertilized in pond water that contains low [Na + ]. The equilibrium potential for Na + is likely too low for TPC3 to generate a large depolarization. Studies have also implicated ulAPs in the oocyte maturation process when the cells are exposed to bodily fluids containing >100 mM Na + (ref. 50 ). However, we did not observe an obvious inhibition of progesterone-induced maturation of X. laevis oocytes treated with 5 μM verapamil, which effectively blocked xlTPC3. Depolarizations similar to the TPC3-mediated one may have functions besides in reproduction. For example, prolonged depolarizations induced by cell damage have been suggested to aid in wound repair and tissue regeneration, which have been characterized in non-mammals that have a higher regenerative capability than mammals [51] . In addition, an EST (expressed sequence tag) database search suggests that the dog TPC3 (accession # XM_005630075) is also expressed in brain (# CO590579), omentum smooth muscle (accession # HS091858) and aorta (# CO671199). The discovery of TPC3 in systems that are amenable to genetic manipulation (for example, zebrafish) allows these hypotheses to be further tested. High-amplitude ulAPs do not appear to be present in all animals. For example, in oocytes and eggs from several mammalian species, such as the mouse, a depolarizing current only elicits APs that last <1 s, presumably resulting from Ca V s. These cells also lack TPC3-like currents [52] , [53] , [54] . The tpc3 gene is found in sea urchins, fish, reptiles, amphibians, birds, cats and dogs, but it is not present in other mammals, such as humans and mice [32] , [33] . The absence of functional tpc3 could explain the apparent lack of ulAPs in some mammals. Future comparative physiological studies with organisms from different kingdoms/phyla will determine whether differences in the presence of the tpc3 gene in the genome are related to differences in behaviour (for example, animal posture) and cellular responses (for example, tissue regeneration and stress responses). Cell culture Animal-use protocols were approved by the Institutional Animal Care and Use Committee at the University of Pennsylvania. Mammalian cells were cultured in a humidified CO 2 (5%) incubator at 37 °C. HEK293T cells (from ATCC) were maintained in Dulbecco's modified Eagle's medium (Gibco) supplemented with 10% fetal bovine serum (Lonza) and 1 × Glutamax (Gibco). Mouse hippocampal neurons were cultured as previously described [55] . Hippocampi were dissected out from P0 pups, chopped into small pieces in ice-cold Ca 2+ -free Hank's balanced salt solution, and digested in Ca 2+ -free Hank's balanced salt solution containing 20 units ml −1 papain and 1 mM L- cysteine hydrochloride for 30 min at 37 °C. Neurons were dissociated by pipetting up and down with a 1-ml tip and plated onto poly-lysine-coated coverslips. In the 24 h after platting, neurons were cultured in Dulbecco's modified Eagle's medium (Biowhittaker) supplemented with 10% Ham’s F-12 (Biowhittaker), 10% bovine calf serum (iron supplemented, Hyclone) and 0.5 × Pen/strep (Gibco). Thereafter the medium was changed to Neurobasal A (Gibco) supplemented with 1 × B-27 (Gibco), 1 × Glutamax and 0.5 × Pen/strep. Transfections were done using Lipofectamine 2000 or Lipofectamine LTX (Invitrogen). Xenopus laevis oocytes (defolliculated with collagenase treatment) were maintained in ND96 solution [56] containing (in mM): 96 NaCl, 2 KCl, 1 MgCl 2 , 1.8 CaCl 2 , 5 HEPES, pH 7.4 (adjusted with NaOH) and 50 μg ml −1 gentamycin, at 19±1 °C. Stage V and VI oocytes were selected for experiments. Each oocyte was injected with 50 nl cRNA (10 ng) or H 2 O using a Nanoject II microinjector (Drummond), and was recorded 2–7 days after injection. Cloning of zebrafish and Xenopus TPCs Full-length Zebrafish, D. rerio , TPCs (drTPC2, drTPC3) and Xenopus laevis TPC3 (xlTPC3) cDNAs were amplified with PCR using first-strand cDNA synthesized from whole-zebrafish ovary or Xenopus oocytes. The forward and reverse PCR primers containing cloning sites had the following sequences: drTPC2 (forward, 5′- TAGTCGACATGGAAGAAGAACCGCTGCTGGCTGGC -3′; reverse, 5′- TACCCGGGTAATTATGTATTAAAGGCCGAGGTGAGGG -3′), drTPC3 (forward, 5′- TAGTCGACATGTCTGAGGGGAAGACTGAGAAAACTAGC -3′; reverse, 5′- TACCCGGGTTATACGGAATCAAAAACAGGGTTTGAGAAGTTGG -3′), xlTPC3 (forward, 5′- ATGGTACCATGTCAGAAGCTGAAGTCACAAGTAATG -3′; reverse, 5′- TGGATCCACTGTAGTTCAACACACCGCCCCAATG -3′). All the clones were completely sequenced to ensure no artificially introduced mutation in the open-reading frames. N -terminally GFP-tagged TPCs were cloned into the SalI/XmaI sites (drTPC3) or the KpnI/BamHI sites (xlTPCs) of pEGFP-C1. Non-tagged drTPC3 were cloned into the HindIII/EcoRV sites of a pTracer-CMV2-based vector. For cRNA synthesis used for Xenopus oocyte injection, open-reading frames without tags were transferred into pGEM-HE vector, which contains untranslated region sequences from Xenopus β-globin to enhance RNA stability and expression in the oocytes [57] ). cRNAs were synthesized from PCR-generated templates using an mMESSAGE mMACHINE T7 kit (Ambion), precipitated with LiCl and resuspended in RNAse-free H 2 O. Imaging Transfected cells were plated onto glass coverslips, fixed with 2% paraformaldehyde and mounted with Fluoroshield with 4′,6-diamidino-2-phenylindole (Sigma). Images were taken with a laser-scanning confocal microscope (Leica TMRE TCS SL) using a × 63 oil objective. Electrophysiology Recordings were carried out at room temperature using a Multiclamp 700B (Molecular Device) for HEK293T cells and neurons, or a GeneClamp 500B amplifier (Axon) for Xenopus oocytes. A Digidata 1440A (Molecular Device) under the control of pClamp software (Molecular Device) was used for data acquisition. Clampfit (Molecular Device) software was used for data analysis. Liquid junction potentials (LJPs) were corrected for all patch-clamp recordings. Unless otherwise stated, bath solution for whole-cell voltage-clamp recordings with HEK293T cells contained (in mM): 145 Na-methanesulphonate, 5 NaCl, 10 HEPES, 10 glucose, pH 7.4. Pipette solution contained (in mM): 130 Na-methanesulphonate, 2.5 MgCl 2 , 10 HEPES, 10 EGTA, 20 NaOH, pH 7.2 (LJP=0.9 mV). For current-clamp recordings with HEK293T cells ( Fig. 7 ), bath solution contained (in mM): 140 NaCl, 5 KCl, 2 CaCl 2 , 1 MgCl 2 , 10 glucose, 20 HEPES, pH 7.4 by NaOH. Pipette solution contained (in mM): 140 K-gluconate, 4 NaCl, 2 MgCl 2 , 0.39 CaCl 2 , 1 EGTA, 10 HEPES, pH 7.2 by KOH (LJP=15.3 mV). For current-clamp recordings with neurons ( Supplementary Fig. 3 ), bath solution contained (in mM): 150 NaCl, 3.5 KCl, 1 MgCl 2 , 1.2 CaCl 2 , 10 HEPES, 20 glucose, pH 7.4 by NaOH. Pipette solution contained (in mM): 135 K-aspartate, 5 KCl, 5 NaCl, 1 MgCl 2 , 1 EGTA, 4 Mg-ATP, 0.3 Na-GTP, 14 phosphocreatine (di-tris), 10 HEPES, pH 7.2 by KOH (LJP=16.0 mV). Whole-endolysosome recordings were performed with enlarged endolysosomes from HEK293T cells treated with vacuolin-1 (1 μM, overnight) as previously described [25] . Bath solution used for endolysosomal recordings contained (in mM): 140 Na-gluconate (or K-gluconate for Supplementary Fig. 2 ), 4 KCl (or NaCl for Supplementary Fig. 2 ), 2 MgCl 2 , 0.39 CaCl 2 , 1 EGTA, 10 HEPES, pH 7.2 by NaOH (or KOH for Supplementary Fig. 2 ). Pipette solution contained (in mM): 145 NaCl, 5 KCl, 1 MgCl 2 , 2 CaCl 2 , 10 glucose, 10 HEPES, 10 MES, 10 glucose, pH 4.6 (adjusted with HCl; LJP=−15.9 mV for Supplementary Fig. 2 ; LJP=−12.5 mV for the others.). The voltage dependence of channel activation was studied with voltage-step protocols (illustrated in Fig. 2a ) using bath and pipette solutions containing 150 mM Na + as the major cation. The activation curve ( Fig. 2e ) was fitted with Boltzmann equation: where G is the conductance, V 1/2 is the half maximum activation voltage, V is the testing voltage and κ is the slope factor. The pipette solution used to determine the relative permeability P Na / P Cs consisted of (in mM) 150 CsOH, 2.5 MgCl 2 , 10 HEPES, 10 EGTA, pH 7.2 by methanesulphonic acid. The bath solution contained (in mM) 50 Na-methanesulphonate, 100 NMDG, 5 HCl, 10 HEPES, 10 glucose, pH 7.4 by methanesulphonic acid (LJP=11.4 mV). The pipette solution used to determine the relative permeability of P Na / P K consisted of (in mM) 140 K-gluconate, 10 KOH, 2.5 MgCl 2 , 10 TEA, 10 EGTA, 10 HEPES, pH 7.2 by methanesulphonic acid. The bath solution contained (in mM) 50 Na-methanesulphonate, 90 NMDG, 10 TEA, 5 HCl, 10 HEPES, 10 glucose, pH 7.4 by methanesulphonic acid (LJP=17.3 mV). The relative permeabilities of TPC3 ( Fig. 4 ) were calculated using the following equations: where E rev is the reverse potential, F is Faraday's constant, R is the gas constant and T is the absolute temperature. We recorded no appreciable current when Ca 2+ was used as the bath cation, indicating that Ca 2+ is impermeable ( Fig. 4a ). We did not calculate P Ca / P Cs because the current was too small to obtain a reversal potential that was not significantly contaminated by the endogenous HEK293 cell currents. We also used Ca 2+ as the major cation in the pipette and Na + in the bath in an attempt to obtain P Na / P Ca ; however, for reasons to be determined, high [Ca 2+ ] in the pipette abolished the depolarization-activated inward Na + current, making it difficult to determine the accurate reversal potential for permeability calculation. The inhibition curves presented in Fig. 5 ; Supplementary Figs 4 and 6 were fitted with the Hill equation: where I and I 0 are the current amplitudes obtained in the presence and absence of channel blockers, respectively, X is the blocker concentration, IC 50 is the concentration required for half-maximal inhibition and h is the Hill coefficient. For two-electrode voltage-clamp recordings with Xenopus oocytes, ND96 was used as the bath solution. Pipettes were filled with 3 M KCl. In an attempt to knockdown xlTPC3 in Xenopus oocytes, we injected an antisense morpholino oligo against xlTPC3, but did not find obvious reduction of the native current, perhaps because of the current’s already small size (~0.3 μA whole cell), the presence of two copies of xlTPC3 genes with differing sequences (not shown) from the tetraploid genome and/or a long lifetime of xlTPC3’s mRNA or protein. Data analysis Data were analysed using Clampfit (Molecular Device), Excel (Microsoft) and OriginPro (Origin lab) and plotted using OriginPro. Numeric data were shown as mean±s.e.m. How to cite this article: Cang, C. et al . A non-inactivating high-voltage-activated two-pore Na + channel that supports ultra-long action potentials and membrane bistability. Nat. Commun. 5:5015 doi: 10.1038/ncomms6015 (2014).